The fidelity of the ligation step determines how ends are resolved during nonhomologous end joining Nonhomologous end joining (NHEJ) can effectively resolve chromosome breaks despite diverse end structures; however, it is unclear how the steps employed for resolution are determined. We sought to address this question by analysing cellular NHEJ of ends with systematically mispaired and damaged termini. We show NHEJ is uniquely proficient at bypassing subtle terminal mispairs and radiomimetic damage by direct ligation. Nevertheless, bypass ability varies widely, with increases in mispair severity gradually reducing bypass products from 85 to 6%. End-processing by nucleases and polymerases is increased to compensate, although paths with the fewest number of steps to generate a substrate suitable for ligation are favoured. Thus, both the frequency and nature of end processing are tailored to meet the needs of the ligation step. We propose a model where the ligase organizes all steps during NHEJ within the stable paired-end complex to limit end processing and associated errors. DNA double strand breaks (DSBs) arise spontaneously, after exposure to DNA-damaging agents, and are also normal intermediates in meiosis and V(D)J recombination. If misrepaired or unrepaired they can lead to cellular cytotoxicity and premature cellular senescence, and at the organismal level developmental defects—including immunodeficiency and neurodegeneration—as well as a predisposition to cancer (reviewed in, for example, ref. 1 ). A robust nonhomologous end joining pathway (NHEJ) is essential for mitigating these defects, but is considered error-prone. This pathway begins with the recognition of broken ends by the Ku heterodimer (Ku70 and Ku80). Ku subsequently recruits the DNA-dependent protein kinase catalytic subunit (DNA-PK CS ) as well as a ligase complex. The ligase complex includes the DNA ligase IV (LIG4) catalytic subunit, as well as XRCC4 and the XRCC4-like factor (XLF/Cernunnos; reviewed in ref. 2 ). The only essential step in NHEJ is the rejoining of at least one strand of the double strand break, via ligation of 5′ phosphate and 3′ OH strand break termini. However, DSBs in vivo often have complex ends, where the structure of aligned ends does not allow for straightforward juxtaposition of strand break termini. Examples include ends with damaged and adducted nucleotides, as well as mispairs, gaps, hairpins and flaps. In vitro studies have determined that the ligation step in NHEJ can remain active even with difficult-to-align termini [3] , [4] , [5] , [6] , [7] , and further identified XLF as important co-factor in facilitating the ability to ligate such ends [8] , [9] . However, the full extent of flexibility of the ligation step in bypassing terminal distortions has not been systematically characterized. It is especially unclear how significant the ability to directly ligate complex ends is in the context of cellular NHEJ, and if bypass is significantly more effective for classically defined NHEJ, relative to other end joining pathways (Alt-NHEJ). Ends can also be processed by a variety of polymerases and nucleases before ligation, in yeast (for example, refs 10 , 11 , 12 , 13 ) and in mammalian models (for example, refs 14 , 15 , 16 , 17 , 18 , 19 , 20 , 21 , 22 , 23 ), and much progress has been made in identifying and characterizing these activities. Products of cellular NHEJ are often associated with extensive heterogeneity, for example, those generated during V(D)J recombination [24] , and after sustained expression of targeted endonucleases (for example, I-Sce I, CRISPR or TALEN; for example, refs 25 , 26 ). This heterogeneity has led to characterization of NHEJ as error-prone, with a stochastic component contributing both to whether ends are processed before ligation, as well as how. Ends can thus be resolved either by direct ligation, bypassing the need for processing, or processed first, but how well the initial structure of an aligned end-pair determines the balance between these two alternatives is still unresolved (reviewed in refs 27 , 28 , 29 , 30 ). Here we address this question with a series of substrates that systematically increases the predicted barrier to ligation in increments and determine in cells how this has an impact on the balance between low-fidelity ligation of a pair of ends versus ligation of these ends after they have first been processed. Our results outline the extent to which NHEJ’s ligation step is capable of bypassing mispairs and damage, and indicates that the path to resolution employed during NHEJ is well-tailored to the needs of different substrates. Substrates to assess the significance of ligation fidelity to NHEJ A series of substrates was designed to investigate how the path to resolution in NHEJ is influenced by gradually increasing the barrier to the ligation step. Each substrate has partly complementary overhangs that generate terminal mispairs (for example, G:T in Fig. 1a i,b ) when aligned. The complementary portion of the overhang was then kept constant for different substrates, and only the terminal mispair varied; for example, 3′ terminal G:T versus G:A as noted in Fig. 1b,c . All substrates can thus be resolved in one step by a ligation (termed direct ligation or bypass) as described in Fig. 1ai . 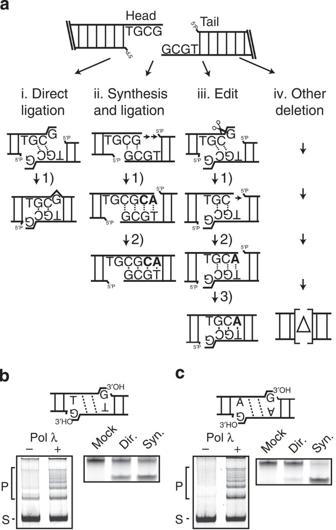Figure 1: Design of substrates. (a) Substrate TGCG3′ is shown; this and related substrates all possess symmetric head and tail end structures that can be aligned to allow for resolution by (i) direct low-fidelity ligation of a terminal mispair, (ii) gap fill-in synthesis and ligation, (iii) excision of the terminal mispair, gap fill-in synthesis and ligation (edit) or (iv) other deletions. Nucleotides added during resolution are bolded. (b) Left panel: TGCG3′ overhang substrate (generates G/T mispair; S) was incubated with Ku, XLF, XRCC4-LIG4 complex and with and without Pol λ (left panel) to generate concatemer ligation products (P). Right panel: junctions were characterized by amplification and mock digested or digested with restriction enzymes diagnostic for direct ligation (Dir.) or synthesis and ligation (Syn.;Supplementary Fig. 1a). (c) A substrate with AGCG3′ overhangs (generates G/A mispair) analysed as inb). Figure 1: Design of substrates. ( a ) Substrate TGCG3′ is shown; this and related substrates all possess symmetric head and tail end structures that can be aligned to allow for resolution by (i) direct low-fidelity ligation of a terminal mispair, (ii) gap fill-in synthesis and ligation, (iii) excision of the terminal mispair, gap fill-in synthesis and ligation (edit) or (iv) other deletions. Nucleotides added during resolution are bolded. ( b ) Left panel: TGCG3′ overhang substrate (generates G/T mispair; S) was incubated with Ku, XLF, XRCC4-LIG4 complex and with and without Pol λ (left panel) to generate concatemer ligation products (P). Right panel: junctions were characterized by amplification and mock digested or digested with restriction enzymes diagnostic for direct ligation (Dir.) or synthesis and ligation (Syn. ; Supplementary Fig. 1a ). ( c ) A substrate with AGCG3′ overhangs (generates G/A mispair) analysed as in b ). Full size image The ends of these substrates can also be processed before ligation, allowing assessment of the extent to which engagement of end processing is responsive to different barriers (that is, mispairs or damage) to the ligation step. However, to address whether the exact nature of end processing could also be influenced by initial end structure, all substrate variants allow for a second alignment that generates a two-nucleotide gap, and which requires only fill-in synthesis before ligation ( Fig. 1a ii ). This latter possibility was intended as an alternate path that is intermediate in complexity between direct ligation ( Fig. 1a i ) and paths where the end is first remodelled by a nuclease step, including resolution by ‘editing’ ( Fig. 1a iii,iv ; discussed in greater detail below). The utility of these substrates was first tested in vitro , using an example with TGCG3′ overhangs. Direct ligation of this substrate would require ‘bypass’ of a G:T 3′mispair, as depicted in the cartoon panel of Fig. 1b . The substrate was incubated with purified Ku, XRCC4-LIG4 complex, XLF and DNA polymerase λ; thus, only two of the paths described in Fig. 1a —ligation or synthesis and ligation—are possible ( Fig. 1a i,ii ). Head-to-tail ligation products were then characterized by digestion of amplified products with restriction enzymes that are diagnostic for each path ( Supplementary Fig. 1a ). A total of 33% of TGCG3′ ligation products were formed via direct ligation, with the remainder attributable to synthesis and ligation ( Fig. 1b , right panel). Omission of either the polymerase or synthesis precursors reduced joining efficiency ( Fig. 1b , left panel; Supplementary Fig. 1b ), indicating direct joining with a G:T 3′ terminal mispair is unable to fully compensate for the absence of a possible synthesis-dependent resolution. NHEJ’s ligase complex is thus only partly able to bypass this mispair. Moreover, only trace levels of joining were observed when T4-DNA ligase was substituted for the XRCC4-LIG4 complex, whether the polymerase was included or not ( Supplementary Fig. 1c ). Therefore, ligase activity per se , i.e., as provided by T4 ligase, was not sufficient for either of the resolutions mediated by the XRCC4-LIG4 complex (bypass of the terminal mispair by direct ligation or polymerase-dependent resolution). The ability of ligases to tolerate mispairs can depend on how similar the mispair width (for example, C1′–C1′ distance) is to that of matched base pairs [31] . We therefore substituted the G:T purine:pyrimidine mispair with the bulkier G:A purine:purine mispair (AGCG3′; Fig. 1c ). Although overall ligation was comparable ( Fig. 1b cf . Fig. 1c , left panels), the proportion of direct ligations was reduced to 4% with this substrate ( Fig. 1c , right panel), with the fraction of synthesis-dependent resolutions increasing to compensate. Accordingly, there was less joining of AGCG3′ than was observed with TGCG3′ when polymerase λ was omitted ( Fig. 1b cf . Fig. 1c , left panels). These substrates thus identify a variable ability of NHEJ to bypass terminal mispairs consistent with previously described patterns of ligase fidelity, and show how a specific processing-dependent resolution path is engaged as a compensating mechanism. Ability of cellular NHEJ to bypass terminal mispairs Is there a similar balance between low fidelity ligation and end processing in cellular NHEJ? In addition, NHEJ in cells employs a variety of processing enzymes—including nucleases—in addition to polymerase activity; thus, ends may be processed by diverse means. These DNA substrates were consequently introduced into a human cell line (HCT 116), and joining was characterized both in terms of efficiency, by quantitative PCR (qPCR) of head-to-tail products, as well as product structure, by sequencing ( Fig. 2a and Supplementary Fig. 2 ). We used conditions that resulted in a rate and capacity of substrate joining comparable to that observed for chromosomal repair after 2 Gray of ionizing radiation ( Supplementary Fig. 3a and Methods). Joining of all substrates under these conditions was primarily mediated by classically defined NHEJ, as reflected by the >10-fold defect in joining efficiency observed in LIG4 −/− cells [32] relative to its isogenic matched wild-type parent ( Fig. 2b ). We additionally confirmed that a diverse product spectrum was maintained through the amplification and sample processing steps required for sequencing analysis ( Supplementary Fig. 2d ). 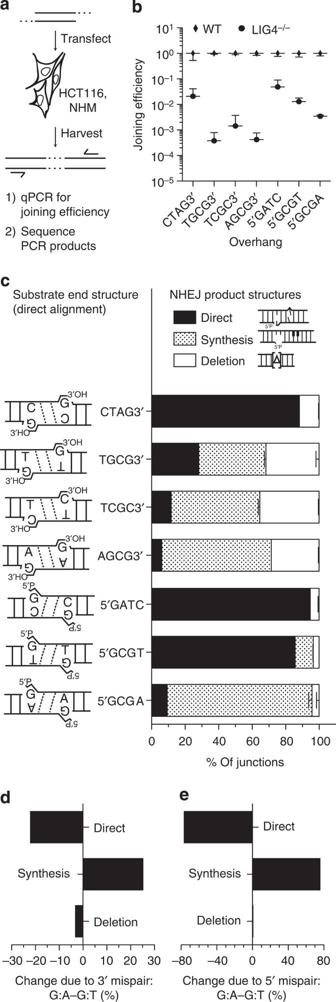Figure 2: Cellular assay for NHEJ of systematically varied end structures. (a) Description of cellular assay. (b) Joining efficiencies for each substrate, comparing wild-type HCT 116 cells to its LIG4-deficient variant (LIG4−/−). Error bars denote the s.d. for 12 (5′GATC, 5′GCGT) or six (all others) independent electroporations. (c) Substrates possessed end structure varied as shown. Product structures were defined as inFig. 1a, and the proportion (%) of each determined by sequencing of junctions from wild-type cells, averaged from two libraries, each library from a pool of three electroporations (see also Methods). Error bars represent the range of results from the two libraries. (d,e) The change in proportion of each resolution path due to differing terminal mispairs was calculated by subtracting the mean proportions for each category of product, first (d)TGCG3′ (3′ G:T) from AGCG3′ (3′ G:A), then (e) 5′GCGT (5′G:T) from 5′GCGA (5′ G:A). Figure 2: Cellular assay for NHEJ of systematically varied end structures. ( a ) Description of cellular assay. ( b ) Joining efficiencies for each substrate, comparing wild-type HCT 116 cells to its LIG4-deficient variant (LIG4 −/− ). Error bars denote the s.d. for 12 (5′GATC, 5′GCGT) or six (all others) independent electroporations. ( c ) Substrates possessed end structure varied as shown. Product structures were defined as in Fig. 1a , and the proportion (%) of each determined by sequencing of junctions from wild-type cells, averaged from two libraries, each library from a pool of three electroporations (see also Methods). Error bars represent the range of results from the two libraries. ( d , e ) The change in proportion of each resolution path due to differing terminal mispairs was calculated by subtracting the mean proportions for each category of product, first ( d )TGCG3′ (3′ G:T) from AGCG3′ (3′ G:A), then ( e ) 5′GCGT (5′G:T) from 5′GCGA (5′ G:A). Full size image The panel of substrates was also expanded to obtain a more comprehensive picture of the contribution of low-fidelity ligation to NHEJ. Substrates with fully complementary overhangs (no terminal mispair) were added to assess the background of end processing observed when there is no barrier to ligation. An end structure with a terminal pyrimidine:pyrimidine mispair (C:T) was also included (TCGC3′). Finally, parallel versions of these 3′ overhang substrates with opposite overhang polarity (5′) were generated. As expected, a fully complementary 3′ overhang was rarely processed before ligation; 88% of the recovered sequences were products of direct ligation when using the CTAG3′ substrate ( Fig. 2c , Supplementary Table 1 ). Directly ligated product then accounted for 28% of recovered sequences for the TGCG3′ substrate (G:T mispair), 12% for TCGC3′ (C:T mispair) and 6% for AGCG3′ (G:A mispair; Fig. 2c ). The proportion of directly ligated product was thus reduced upon inclusion of a mispair, and then reduced further with increasing predicted severity of the terminal mispair (see Supplementary Table 2 for statistical analyses of significance). The proportions of direct joining observed for TGCG3′ and AGCG3′ during cellular NHEJ were also similar to the proportions observed in in vitro reactions with these substrates ( Fig. 1b,c ). A similar progressive reduction in direct ligation was observed for the panel of 5′ overhangs, from 94% (5′GATC; paired) to 85% (5′GCGT; G:T mispair) to 9% (5′GCGA; G:A mispair; Fig. 2c ). However, mispairs at the terminus of a 5′ overhang were more easily tolerated than the comparable mispair at the terminus of a 3′ overhang ( P <0.0001, Supplementary Table 2 ). This was most apparent for the G:T mispair, where directly ligated products were threefold more frequent when the mispair was within a 5′ overhang, relative to a 3′ overhang. Cellular NHEJ thus favours direct ligation of terminal mispairs (ligation ‘bypass’) when possible. Effects of terminal mispairs on end processing If ends cannot be ligated directly, there is great flexibility in how they can be processed during cellular NHEJ—any of the paths described in Fig. 1a could be employed and chosen at random, leading to heterogeneity in products. Instead, decreasing ability to bypass different terminal mispairs in different substrates typically resulted in progressively increased recovery of the single junction sequence that is indicative of synthesis and ligation ( Figs 1a ii , 2c ; Supplementary Table 2 ). Strikingly, the redirection of resolution path was often seamless; reduction in ability to resolve by direct ligation often resulted in a near-equal increase in resolution by synthesis and ligation (for example, Fig. 2d,e ). When assessing synthesis, substitution error at sites of cellular polymerase activity was less than 2 × 10 −3 , and indistinguishable from that attributable to sample processing ( Supplementary Fig. 3b ). In addition, both nucleotides of the two-nucleotide gaps were usually (>98%) filled-in ( Supplementary Fig. 3c,d ). Resolutions associated with deletion were typically rare. For the majority of substrates, we recovered over 40 different junction sequences with terminal sequence deleted, but they accounted for in sum 12% or less of products ( Fig. 2c ). Substrates that both had 3′ overhangs and can align with a terminal mispair were the exception: resolutions after deletion were over twice as frequent for this class of substrates, relative to any other substrate ( Fig. 2c ). The observed increase in deletions was further largely limited to a specific kind of deletion, where the sequence lost was restricted to one or both of the single stranded DNA overhangs (ssDNA deletion; Fig. 3a,b ). Therefore, a class of ends that are especially poorly bypassed by direct ligation (3′ terminal mispairs; Fig. 2c ) triggers use of an alternate (third) path for their resolution, where end structure is more generally altered, or remodelled, by activity of a ssDNA endo/exonuclease. Artemis is a likely candidate for this activity [33] , [34] (see also Discussion). 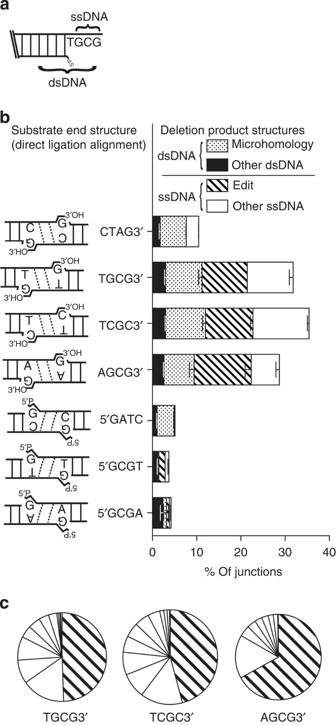Figure 3: Characterization of junctions with deletions. (a) Deletions were categorized according to whether deleted sequence was entirely limited to the single stranded overhangs (ssDNA deletion), then further categorized as whether the junction equaled the ‘edit’ product described inFig. 1a iiiversus all other ssDNA deletions. Similarly, junctions where deleted sequence extended into flanking double stranded DNA (dsDNA deletion) then classed as occurring at a flanking sequence identity (microhomology-mediated) or not (other dsDNA). (b) Proportions of junctions with deletion (Fig. 1a, iii,iv) fromFig. 2cresults were further categorized as in (a). Error bars represent the range of results from the two libraries. (c) The area of each slice is representative of the proportion of a different junction sequence with ssDNA deletion, as a fraction of the total sequences with ssDNA deletion (Fig. 3a,Supplementary Table 3). The proportion of edits (Fig. 1a iii) is distinguished from deletions not guided by overhang sequence complementarity. Figure 3: Characterization of junctions with deletions. ( a ) Deletions were categorized according to whether deleted sequence was entirely limited to the single stranded overhangs (ssDNA deletion), then further categorized as whether the junction equaled the ‘edit’ product described in Fig. 1a iii versus all other ssDNA deletions. Similarly, junctions where deleted sequence extended into flanking double stranded DNA (dsDNA deletion) then classed as occurring at a flanking sequence identity (microhomology-mediated) or not (other dsDNA). ( b ) Proportions of junctions with deletion ( Fig. 1a, iii,iv ) from Fig. 2c results were further categorized as in ( a ). Error bars represent the range of results from the two libraries. ( c ) The area of each slice is representative of the proportion of a different junction sequence with ssDNA deletion, as a fraction of the total sequences with ssDNA deletion ( Fig. 3a , Supplementary Table 3 ). The proportion of edits ( Fig. 1a iii ) is distinguished from deletions not guided by overhang sequence complementarity. Full size image Notably, the most frequent junction with overhang-limited deletion (ssDNA deletion; Fig. 3c , Supplementary Table 3 ) can be readily explained as a product of a path that is also alignment-directed and employs only a single extra step, relative to the other paths already discussed. Editing ( Fig. 1a iii ) requires (1) removal of the terminal nucleotide by a nuclease, (2) alignment of the remaining overhang and fill in of the resulting one-nucleotide gap by a polymerase, followed by (3) ligation. Consistent with this inferred three-step pathway, the recovery of the edit product, as well as most of the other deletions, are severely reduced in cells deficient in both NHEJ polymerases (Pol μ and Pol λ; C.A.W., J.M.P. and D.A.R, unpublished data). Inasmuch as this resolution path involves replacement of a terminal mispair with a complementary nucleotide, it is analogous to the editing of terminal mispairs after polymerase misincorporation (see also the Discussion, below). Editing is guided by alignment of the same amount (2 bp) of complementary sequence in the overhangs as the previously discussed paths ( Fig. 1a ), and thus can be considered equally favourable. Editing is consequently distinguished from ‘other deletions’ in subsequent figures. This is also rationalized by the observation that other deletions can be slower to accumulate than junctions with editing, as discussed below ( Fig. 4b,c ). 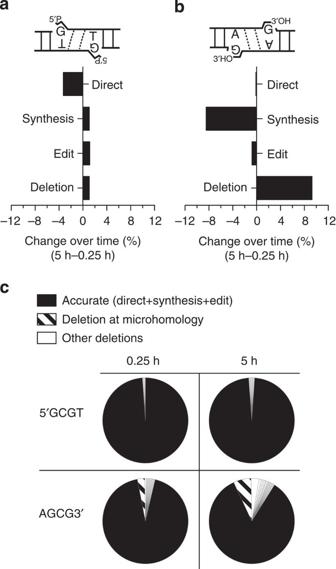Figure 4: Changes in resolution path over time in the cell. (a,b) The change in proportion (%) of resolution path, comparing product recovered 5 h versus 15 min in cells, for 5′GCGT (a) and AGCG3′ (b). (c) The frequency of different junctions, distinguishing accurate (filled section), microhomology-directed deletions (diagonal bars), and all other deletions (open sections) for 5′GCGT versus AGCG3′ substrates, after 15 min versus 5 h in cells. Figure 4: Changes in resolution path over time in the cell. ( a , b ) The change in proportion (%) of resolution path, comparing product recovered 5 h versus 15 min in cells, for 5′GCGT ( a ) and AGCG3′ ( b ). ( c ) The frequency of different junctions, distinguishing accurate (filled section), microhomology-directed deletions (diagonal bars), and all other deletions (open sections) for 5′GCGT versus AGCG3′ substrates, after 15 min versus 5 h in cells. Full size image Deletions that extended into flanking double stranded DNA (dsDNA deletions) were in total rare, although deletions guided by fortuitous sequence identities (microhomologies; Figs 3a,b and 4c ) were enriched among these, as has been previously observed [14] . Changes in resolution path over time We describe above how the identity of a terminal mispair affects the balance between direct ligation versus ligation after end processing, and were interested in determining whether this balance changes over time. Products were therefore recovered after 15 min in cells and results compared with our previous data, where the products were recovered after 5 h. This comparison was performed using both a substrate (5′GCGT) that favours resolution by direct ligation, as well as a substrate (AGCG3′) that favours a resolution path requiring a processing step. Resolution paths for 5′GCGT ends changed very little with prolonged time in cells ( Fig. 4a ). In contrast, the primary mechanism for resolution of AGCG3′ ends—synthesis and ligation—decreased over time (8.5%), with deletions increased to compensate ( Fig. 4b ). Resolutions by synthesis and ligation were thus surprisingly under-represented upon extended incubation, even when compared with resolutions by direct ligation. We conclude the need to perform an additional enzymatic step (synthesis) was not rate-limiting, at least for this substrate. As noted above, direct ligation, synthesis and ligation, and editing are all guided by the same amount of complementary sequence in the overhang, and are thus equally favoured ( Fig. 1a ). Together, they account for the clear majority of products after 15 min in cells for both substrates (99 and 94% for 5′GCGT and AGCG3′, respectively; Fig. 4c ). Remaining products were associated with greater amounts of deleted sequence, and included both heterogeneous and microhomology-determined products. This less accurate class was initially rare and increased slowly, although rates differed depending upon substrate. Importantly, the limited product heterogeneity observed even for the 15-min sample was not a function of sampling error. An equivalent number of input template molecules (determined using qPCR) were used for all four libraries for each substrate (two replicates of each timepoint), as well as the library that validated ability to sample diverse product spectra ( Supplementary Fig. 2d ). Changes in resolution path in different cell types To discern to what extent our results were specific to the HCT 116 cell line, we next assessed how these substrates were resolved by performing parallel experiments with selected substrates in a primary human melanocyte culture (passage 8; Fig. 5a ). The trends in mispair tolerance were the same for melanocytes as in HCT 116 cells; direct joining was more frequent for a pyrimidine:purine mispair, relative to a purine:purine mispair (93% for 5′GCGT cf . 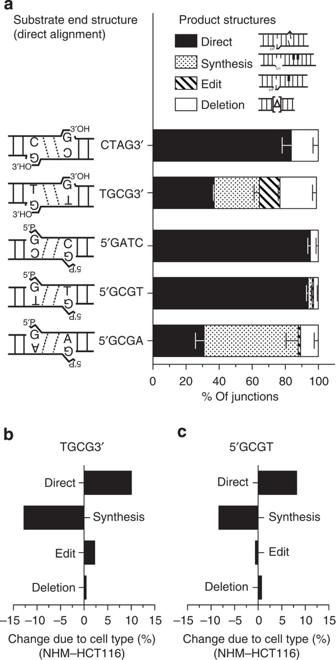Figure 5: NHEJ of systematically varied end structures in melanocytes. (a) Selected substrates were introduced into melanocytes (NHM) and characterized as described inFig. 2c, except results are from three independent libraries (nine electroporations). (b,c) The change in proportion of each resolution path comparing NHM and HCT116 cells for substrates TGCG3′ (b) and 5′GCGT (c). 30% for 5′GCGA; Fig 5a , P <0.0001; Supplementary Table 2 ). The same mispair was also better tolerated in the context of 5′ overhangs, relative to 3′ overhangs (93% for 5′GCGT cf . 37% for 3′GCGT; Fig 5a , P <0.0001; Supplementary Table 2 ). Figure 5: NHEJ of systematically varied end structures in melanocytes. ( a ) Selected substrates were introduced into melanocytes (NHM) and characterized as described in Fig. 2c , except results are from three independent libraries (nine electroporations). ( b , c ) The change in proportion of each resolution path comparing NHM and HCT116 cells for substrates TGCG3′ ( b ) and 5′GCGT ( c ). Full size image In contrast, cell type significantly altered the balance between resolution paths for a given substrate. Bypass or direct ligation of mispairs was more frequently employed in melanocytes, relative to HCT 116 cells, for all three of the substrates with partly complementary overhangs that were tested ( Fig. 5b,c ). As with differing substrate, changes in resolution by direct ligation due to different cell line were primarily compensated for by a change in resolution by the next-most-simple path in terms of numbers of steps (synthesis and ligation). The ability of cellular NHEJ to bypass terminal damage The above experiments focused on strand break termini that interfered with ligation because they were mispaired. Damaged termini may be qualitatively different, and removed regardless of whether they are a significant barrier to ligation. We therefore generated a substrate with a terminal 8-oxo-7,8-dihydroguanine (G O ), the most abundant base damage generated by ionizing radiation [35] and thus expected to be near damage-induced breaks. The overhang was otherwise complementary (5′G O ATC), and consequently this substrate assessed the ability of NHEJ to tolerate a terminal 5′G O :C damaged pair. Wild-type cells were equally able to join 5′GATC (5′G:C paired terminus), 5′GCGT (5′G:T mispaired terminus) and 5′G O ATC (5′G O :C damaged pair terminus; Fig. 6a ). LIG4-deficient cells also retain significant activity on the undamaged, paired terminus (5′GATC), consistent with activity of remaining mammalian ligases. However, LIG4-deficient cells were much less active in joining ends with terminal distortions, especially when considering the Go:C damaged pair (5′G:C cf . 5′G O :C, Fig. 6a ). Joining of ends with the damaged G O :C pair is also specifically and severely reduced in cells deficient in Ku 70 (5′G:C cf . 5′G O :C, Supplementary Fig. 4a ). We conclude that classically defined NHEJ is uniquely effective in joining ends with a terminal G O :C pair. 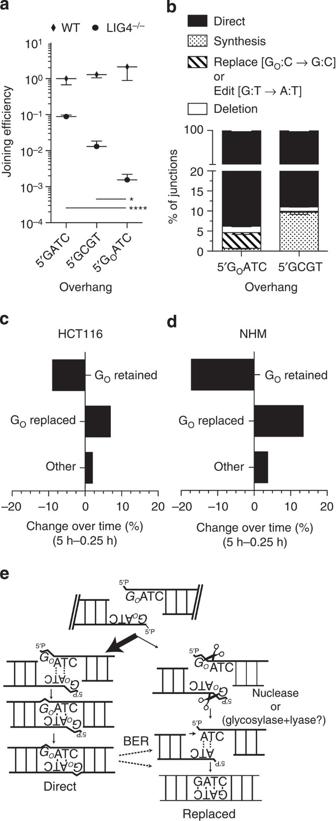Figure 6: NHEJ of ends with a terminal 8 oxoguanine. (a) Joining efficiencies for each substrate and cell line, all compared with joining of undamaged 5′GATC in wild-type cells. Error bars represent the s.d. from six independent electroporations. Joining in LIG4-deficient cells was significantly different for 5GOATC compared with the other two substrates (*P<0.05; ****P<0.0001; one-way analysis of variance comparing results of six independent electroporations for each group, withPvalues adjusted to account for multiple comparisons by the Bonferoni method). (b) The proportion of junctions joined by noted resolution paths in HCT 116 cells after 15 min in cells, averaged from two libraries, each library from a pool of three electroporations. Error bars note the range. (c,d) The change in proportion of each resolution path comparing 5 h versus 15 min, for HCT 116 cells (c) and melanocytes (d). (e) Pathways for replacing GOwith undamaged G. Figure 6: NHEJ of ends with a terminal 8 oxoguanine. ( a ) Joining efficiencies for each substrate and cell line, all compared with joining of undamaged 5′GATC in wild-type cells. Error bars represent the s.d. from six independent electroporations. Joining in LIG4-deficient cells was significantly different for 5G O ATC compared with the other two substrates (* P <0.05; **** P <0.0001; one-way analysis of variance comparing results of six independent electroporations for each group, with P values adjusted to account for multiple comparisons by the Bonferoni method). ( b ) The proportion of junctions joined by noted resolution paths in HCT 116 cells after 15 min in cells, averaged from two libraries, each library from a pool of three electroporations. Error bars note the range. ( c , d ) The change in proportion of each resolution path comparing 5 h versus 15 min, for HCT 116 cells ( c ) and melanocytes ( d ). ( e ) Pathways for replacing G O with undamaged G. Full size image Oxidized nucleotides, especially 8-oxoguanine, can be targeted for removal. We therefore assessed whether we could detect G O in product, to determine whether G O was bypassed by direct ligation (as with G:T mispair) or whether G O was replaced with an undamaged G before ligation. G O in product was estimated by sequencing analysis, as templates with G O generate characteristic transversion mutations [36] after amplification. We further evaluated the frequency of transversion mutation opposite G O in template under our conditions using a model template and employed this frequency as a correction factor (see also Methods). A parallel analysis using an enzymatic probe for G O in the product was generally confirmatory ( Supplementary Fig. 4b,c and Methods). In addition, we note that both approaches underestimate the amount of retained G O , as templates with G O are less efficiently amplified (by a factor of 2 under our conditions) than undamaged templates ( Supplementary Fig. 2b ). Thus, at least 94% of the products retained G O (‘direct ligation’) when recovered after 15 min of incubation in HCT 116 cells ( Fig. 6b ). The frequency of processing for the terminal G O :C pair was comparable to an undamaged terminal G:C pair ( Fig. 2c ), and less than even the most easily bypassed mispair (5′G O ATC cf . 5′GCGT; Fig. 6b ). Of processing events, G O was most frequently replaced with undamaged G, rather than deleted ( Fig. 6b ). Notably, end sequence was designed to also allow for an alternate alignment through two terminal G O ( syn ):A( anti ) base pairs, generating a two-nucleotide gap, but less than 0.1% of recovered products were consistent with resolution after such an alignment. We conclude that NHEJ’s ligation step is highly effective in direct bypass of a terminal 8-oxo-7,8-dihydroguanine. The frequency of G O replacement was increased after 5 h, and was approximately twice as efficient in melanocytes, relative to HCT 116 cells ( Fig. 6c cf . Fig. 6d). It is possible that replacement precedes NHEJ’s ligation step ( Fig. 6e ), similar to editing of terminal mispairs. However, G O :C>G:C replacement in product was significantly delayed ( Fig. 6c ), in contrast to observations for mispair editing (G:T>A:T; Fig. 4 ). We therefore favour a model where replacement of the damaged nucleotide occurs after NHEJ is complete and is mediated by base excision repair. Regardless, such replacement was inefficient—even after incubation for 5 h, over 80% of junctions from HCT 116 cells retained the damaged nucleotide. Classically defined NHEJ is thus effective at directly ligating together ends with 5′ terminal 8-oxo-7,8-dihydroguanine—even though the same substrate severely blocks joining by alternate mammalian ligase(s) and pathways active in cells deficient in LIG4 ( Fig. 6a ) or Ku70 ( Supplementary Fig. 4a ). We assessed here how well the ligation step during NHEJ can bypass terminal distortion during cellular NHEJ, using substrates where terminal distortion was increased in increments. We show that the ligation step during cellular NHEJ is effective in tolerating a variety of terminal mispairs, but especially a damaged base pair, 8-oxo-7,8-dihydroguanine:C (G O :C), expected to be frequent at radiation-induced DSBs ( Figs 2c and 6b ). In contrast, in cells missing either LIG4 ( Fig. 6a ) or Ku70 ( Supplementary Fig. 4a ), joining of ends with terminal G O was reduced over 40-fold relative to the undamaged control substrate. The robust joining sometimes observed in LIG4- or Ku70-deficient cells has been used to define ‘Alt-NHEJ’ [37] , [38] , thus we conclude that DSBs with terminal 8-oxo-7,8-dihydroguanine are extremely poor substrates for this pathway. Our results imply that the LIG4 holoenzyme (LIG4, Ku, XRCC4, XLF) may act effectively as a ‘translesion’ ligase. That is the NHEJ complex could be unique among mammalian ligase machines in its proficiency in ligating a DSB terminus with G O opposite C much as DNA polymerase η is unique among mammalian polymerases in its proficiency in adding A opposite a thymidine dimer [39] . As is the case for translesion polymerases, sustained activity on damaged substrates may rely at least in part on structural elements intrinsic to the enzyme. Consistent with this idea, a structure of LIG4 identified elements predicted to interact with substrate that are unique among mammalian ligases, and argued to be significant in ligation of distorted termini [40] . There was nevertheless a wide range in cellular NHEJ’s bypass ability: when challenged with varied mispairs, the proportion of direct ligations decreased in decrements from 85% (5′G:T mispair) to 6% (3′G:A mispair; Fig. 2c ; Supplementary Table 2 ). Generally, the mispairs that are better tolerated during cellular NHEJ are those with width similar to that of a pyrimidine:purine, and which are 5′ of the strand break. This pattern is consistent with that observed for other eukaryotic ligases in vitro ( Figs 2 and 5 ; see Supplementary Table 2 for statistical tests) [31] , [41] . It is best explained if significant LIG4 activity requires it to fully encircle dsDNA flanking a strand break and primarily engage the 5′ side, as observed in structures of other mammalian ligases [42] , [43] and in DNA-bound models for LIG4 (ref. 40 ). NHEJ’s ligation step is thus far-removed from structure independence. How is the means (or path) for resolving a complex end determined during cellular NHEJ? Past studies show resolution of broken ends by NHEJ is guided by alignment of complementary sequence in overhangs when present [14] ; in this study, they accounted for 75–98% of junctions ( Figs 2c and 3b , Supplementary Table 1 ). The substrates described here were further designed such that each allows for three such alignment-directed resolution paths—direct ligation, synthesis and ligation, and editing—with all three paths guided by an alignment of the same amount of complementary sequence (two nucleotides; Fig. 1a ). Our results thus speak directly to how resolution paths are chosen for different end structures, given initial alignments that are equally favourable. As noted above, ends are resolved by one-step direct ligation when terminal distortion is sufficiently mild. However, as direct ligation is made more difficult, reductions in direct ligation are almost entirely accounted for by increases in the next most-simple resolution, the two-step synthesis and ligation. This is apparent both when comparing different 5′ mispairs ( Fig. 2e ), as well as different 3′ mispairs ( Fig. 2d ). However, there is a consistent difference in how ends are processed when comparing 5′ versus 3′ mispairs; deletion is at least twofold more frequent for substrates of the latter class, regardless of cell type ( Fig. 3b ). We suggest that deletion is important primarily in contexts where both polymerase and ligase activities are either very inefficient or blocked. Such contexts include 3′ mispairs, as described here, but presumably other blocking lesions as well (for example, 3′ phosphoglycolate). Poor tolerance of 3′ mispairs by the other mammalian ligases has been rationalized previously as an advantage in the context of excision repair pathways (base excision and nucleotide excision repair) [44] , as a means to promote ability to proofread or edit the misincorporation errors from an earlier polymerase step. Notably, the most abundant deletion observed for 3′ mispairs is consistent with such a process (edit; Figs 1a and 3b,c ). Thus, increased deletion at 3′ terminal mispairs in NHEJ has a mechanistic basis—as a group they are the least well tolerated by the ligase—but possibly also a biological rationale, as a means for correcting frequent polymerase misincorporation error. We conclude that the mechanism used for resolving mispaired or damaged ends during cellular NHEJ is adapted to the specific aligned end-pair. Our results further argue that this is achieved by giving precedence to resolution paths with the fewest number of enzymatic steps—direct ligation (one step) is favoured over synthesis and ligation (two steps), which is favoured over more complex paths that include deletion (typically one or more excision steps, followed by synthesis and ligation; at least three steps, for example, edit). This organization of resolution path is best explained if there is also a hierarchy in attempted DNA transaction ( Fig. 7 ). Direct ligation is attempted first, and synthesis attempted next if ligation fails, and excision restricted to specific contexts where end structure requires end remodelling. 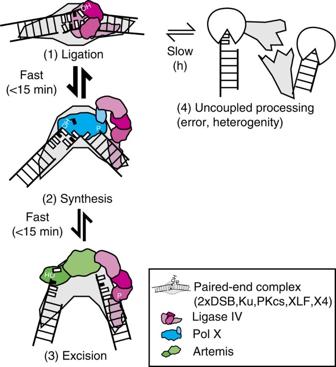Figure 7: Model for organization of enzymatic steps during NHEJ. A model for the order of steps and the configurations of ends and enzymes during repair by NHEJ. Figure 7: Model for organization of enzymatic steps during NHEJ. A model for the order of steps and the configurations of ends and enzymes during repair by NHEJ. Full size image Relative to nucleotide excision repair or base excision repair, where excision is typically followed by synthesis, then ligation (‘cut, copy and paste’; for example, ref. 45 ), this hierarchy of attempted enzymatic step is inverted. An inverted base excision repair analogy may extend to how NHEJ ensures continuity in attempted enzymatic steps. ‘Hand-off’ to the next step in base excision repair is thought to be aided by recognition of the prior step’s enzyme–product complex, rather than simply recognition of free product [45] , [46] . In NHEJ, we have argued the first step is attempted formation of a productive, closed configuration by LIG4 ( Fig. 7 , step 1). We propose that transition to the next step in this pathway involves recognition by end processing enzymes not of a productive enzyme–product complex (as in base excision repair), but of the unproductive, open-configuration LIG4–substrate complex ( Fig. 1 , steps 2 and 3). Such a mechanism is enabled by the tethering of LIG4 to the substrate even in its open configuration, through interactions between its C -terminal domain and a well-discussed DNA–protein ‘splint’ (XRCC4, XLF, Ku and DNA-PKcs) [47] , [48] , [49] . In addition, both X family polymerases [50] and Artemis [51] directly interact with LIG4. An interesting possibility is that these interactions require LIG4 to be in its open configuration. A key role of the ligase in organizing end-processing is further supported by recent studies studying NHEJ with catalytically defective LIG4 (refs 52 , 53 ). Of note, the enzymes that engage ends in successive steps will also dictate discrete changes in how ends are configured, which in turn will allow for sampling of alternate alignments ( Fig. 7 ). Channeling of substrate to different paths due to differing context (substrate, cell type) is efficient ( Figs 2d,e and 5b,c ). This implies that transitions between different steps of multiple-step pathways occur without intervening dissociation of a given end-pair. All three alignment-directed paths are also in total enriched when cellular incubation was limited to 15 min, relative to 5 h ( Fig. 4 ). Taken together, our results imply that accurate NHEJ occurs within a sustained paired-end complex capable of, as needed, rapid and seamless sampling of all three methods for engaging ends and completion of accompanying catalytic steps ( Fig. 7 ). A resolution requiring more steps does not necessarily require more time in the cell to accumulate. Rather, two-step resolutions can accumulate more rapidly than one-step resolutions, when the former resolution path is favoured ( Fig. 4b , cf . Synthesis versus Direct). This is best explained if successive engagements of ends by different enzymes occur within a stable complex, is reversible, and reaches equilibrium within 15 min ( Fig. 7 ). Increasing terminal distortion may make the ligase closed configuration less tenable, which then shifts the equilibrium to promote more frequent interaction of termini with end processing enzymes. This model explains how resolution steps can be easily adapted in graded manner to account for different contexts; most obviously for differing substrate (as discussed above), but also differing availability of end-processing enzymes in different cell types. For example, HCT 116 cells more readily employ synthesis as a compensating mechanism, relative to melanocytes ( Fig. 5b,c ; P <0.0001, Supplementary Table 2 ), possibly due to differences in availability of the X family polymerases implicated in the synthesis step. Heterogeneity and error are derived from a fourth class of products ( Fig. 1a iv). These resolutions accumulate only slowly in the cell and, although not guided by alignment of complementary sequence in the overhang, they include microhomology-mediated junctions (that is, guided by complementary sequence in flanking double stranded DNA; Fig. 4c ). We suggest that these junctions form when processing is uncoupled from the paired end complex ( Fig. 7 , step 4). Processing may have occurred before engagement of ends by the core NHEJ machinery, and/or resolutions may be mediated by another end joining pathway (Alt-NHEJ). The above suggested organization of attempted steps, as well as how well the type of enzymatic step is dictated by initial end structure, contrasts with currently favoured models for NHEJ. We show that the decision whether or how to process complex ends is not stochastically determined, nor is there a threshold of terminal distortion where resolution path discretely switches from direct ligation to processing-dependent resolutions. Resolution path is instead adaptive. Direct ligation is attempted first, to take advantage of a unique effectiveness of the ligation step in NHEJ in bypassing subtle damage at DSB termini. However, we suggest that the ligase can also act effectively as a damage sensor. When damage cannot be easily bypassed by direct ligation, it promotes coupling of failed ligation to an appropriate response, where processing enzymes perform the minimum steps necessary to turn a given aligned end-pair into a substrate that can now be ligated. Substrates and NHEJ assays Substrates were made by amplifying a 300-bp fragment using the primers described and digested with Bsa I or Bst XI to generate the appropriate end structure. In addition, each substrate’s ‘head’ was made identical to that of its ‘tail’ ( Fig. 1a ), ensuring the paths to resolution for all three possible aligned end-pairs (head to head, tail to tail and head to tail) are equivalent. Primer sequences were: CTAG3′: 5′-GTGGTCCACCTAGATGGCTTAGCTGTATAGTCA-3′ 5′-GCCGACCAGCTAGATGGCACACCCATCTCA-3′ TGCG3′: 5′-CAAGTGGTCCACCGCAATGGCTTAGCTGTATAG-3′ 5′-GCCGACCAGCGCAATGGCACACCCATCTCA-3′ TCGC3′: 5′-CAAGTGGTCCACGCGAATGGCTTAGCTGTATAG-3′ 5′-GCCGACCAGGCGAATGGCACACCCATCTCA-3′ AGCG3′: 5′-CAAGTGGTCCACCGCTATGGCTTAGCTGTATAG-3′ 5′-GCCGACCAGCGCTATGGCACACCCATCTCA-3′ 5′GATC: 5′-CAAGTGGTCTCCGATCATCGCTTAGCTGTATAG-3′ 5′-GCCGAGGTCTCAGATCATCACACCCATCTCA-3′ 5′GCGT: 5′-CAAGTGGTCTCCGCGTATCGCTTAGCTGTATAG-3′ 5′-GCCGAGGTCTCAGCGTATCACACCCATCTCA-3′ 5′CGCT: 5′-CAAGTGGTCTCCCGCTATCGCTTAGCTGTATAG-3′ 5′-GCCGAGGTCTCACGCTATCACACCCATCTCA-3′ 5′GCGA: 5′-CAAGTGGTCTCCGCGAATCGCTTAGCTGTATAG-3′ 5′-GCCGAGGTCTCAGCGAATCACACCCATCTCA-3′ 5′G O ATC: 5′-AGTGGTCTCCG O ATCCTCGCTTAGCTGTATAGTCA-3′ 5′-GGTATGTTGGTCTCAG O ATCCTCACACCCATCTCAGAC-3′. Substrates for in vitro assays were labelled by amplification in the presence of αCy5-dCTP (GE Healthcare), and cartridge-purified (Qiaquick PCR Purification, Qiagen). Human Ku, XRCC4-LIG4 complex and XLF were overexpressed in Hi-5 cells. Cell pellets were extracted, lysed by sonification, clarified and loaded on a His-TRAP column (GE Biosciences). Bound protein was eluted by a step-increase to 350 mM imidazole before loading on a Mono-Q column (GE Biosciences) and eluted with a linear gradient of KCl. Fractions encompassing the peak of eluting protein were pooled, flash-frozen in liquid nitrogen and stored at −80 °C (refs 22 , 54 ). Human polymerase λ was purified after expression in bacteria, and was the gift of Dr. Tom Kunkel. In vitro NHEJ reactions were initiated by mixing 10 nM Ku, 20 nM XRCC4-LIG4 complex or 100 units T4 DNA ligase (NEB), 2 nM polymerase and 2 nM DNA substrate in a buffer with 25 mM Tris-Cl (pH7.5), 1 mM dithiothreitol, 150 mM KCl, 4% glycerol, 40 μg ml −1 bovine serum albumin, 0.1 mM EDTA, 7.5% polyethyelene glycol (MW 8,000 kDa), 100 μM of each dNTP, 5 mM Mg 2+ and 100 ng supercoiled DNA. All reactions were carried out at 37 °C for 10 min, stopped by addition of EDTA and SDS, extracted with a 1:1 mixture of phenol and chloroform and resolved on a 5% native PAGE gel. Junctions were characterized by amplification with primers specific for head to tail junctions (5′-CTTACGTTTGATTTCCCTGACTATACAG-3′ and 5′-GCAGGGTAGCCAGTCTGAGATG-3′), and digested with Bst XI as diagnostic for direct joining, and Afe I (AGCG3′) or Fsp I for (TGCG3′) as diagnostic for synthesis and ligation ( Supplementary Fig. 1a ). Digestion products were visualized using a Typhoon Imager and quantified using ImageQuant (GE Healthcare). Except for the 5′G O ATC substrate, substrates used in cellular NHEJ assays were generated by amplification, subcloned into the pCR2.1-TOPO TA vector (Invitrogen) and sequenced. Purified plasmid DNA was then digested using the appropriate restriction enzyme, and the fragment purified by agarose gel electrophoresis. Accuracy of end structures after digestion was further validated at high resolution by visualization of both strands of one end of the substrate in the context of a short (48 bp) subfragment on a denaturing 7% polyacrylamide gel, after serial treatment of gel purified substrate with Hin f1, phosphatase and T4-kinase, in the presence of γ 32 P-ATP ( Supplementary Fig. 2a ). 5′G O ATC was generated as described for in vitro assays, except without αCy5-dCTP label. HCT116 and its LIG4-deficient variants were cultured in McCoy’s 5 A media with 10% fetal calf serum and human melanocyte cells (NHM) cultured in DermaLife M medium (Lifeline Cell Technology). Mouse dermal fibroblasts deficient in Ku70 and p53 were the gift of Dr P. Hasty (UT San Antonio), complemented by expression of mouse Ku70 cDNA or empty vector (pBABE-puro) and grown in Dulbecco’s Modified Eagle Medium with 10% fetal calf serum and 2 μg ml −1 puromycin. A total of 20 ng of the purified, validated substrate and 600 ng of pMAX-GFP (green-fluorescent protein) were introduced into 2 × 10 5 of these cells by electroporation (Neon, Life Technologies) using a 10-μl chamber and one 1530 V, 20 ms pulse (HCT116); three 1,500 V, 10 ms pulses (NHM); or one 1,350 V, 30 ms pulse (Ku70 −/− ), then incubated in 300 μl of the appropriate media without antibiotic at 37 °C for 5 h or 15 min as indicated. Under these conditions 81% (±4%) of HCT116 cells express GFP and 88% (±3.6%) exclude propidium iodide after 5 h, with results indistinguishable for both parental cells and LIG4 −/− variants. Electroporations were performed in triplicate, then repeated in triplicate for each substrate and cell line pair on a second day. A single electroporation (out of the 138 analysed in Figs 2 and 6 ) was excluded from analysis because of failed electroporation or sample loss during recovery. Cells were then washed with phosphate-buffered saline before harvesting of total cellular DNA (QIAmp, Qiagen) except for the experiment described in Supplementary Fig. 3a , where cells had to be lysed without washing. Junctions in recovered DNA were assessed by quantitative real-time PCR, using an ABI 7900HT (Applied Biosystems), primers that amplify head-to-tail junctions (see above), and SYBR green detection. These primers will amplify junctions having deletions up to 13 and 12 nucleotides from left and right flanks, respectively (25 nucleotides total) for 5′ overhang containing ( Bsa I generated) substrates. For 3′ overhang substrates we added an additional two nucleotides in the right flank to allow for inclusion of the Bst XI site; the same primers thus amplify junctions up to 27 nucleotides for these substrates. Previous work indicates that this is sufficient to sample products generated by canonically defined NHEJ (for example, refs 26 , 55 ). We validated amplification efficiency and ensured that quantification was performed in a linear range by including a standard curve ( Supplementary Fig. 2b ) in parallel with experimental samples. The standard curve was generated by serially diluting an oligonucleotide model amplicon (product of 5′GATC substrate) into DNA harvested from a mock transfection. We estimate, using serial harvests after electroporation, that joining accumulated to a maximum within an hour ( Supplementary Fig. 3a ). Using the standard curve we further estimated the average accumulation of product molecules for all 5-h experiments in HCT 116 cells described here was 60 per cell (s.e.m.±6.1). Additional experiments indicated product increases proportionately with increased substrate; thus, repair capacity was not saturated under these conditions. We conclude that the rate and capacity of NHEJ measured here is comparable to that observed for repair of chromosome breaks after exposure of cells to 2 Gray of ionizing radiation [56] , [57] . In Fig. 2 we limit analysis to pairwise comparison of joining efficiencies in wild type versus LIG4-deficient cells for each individual substrate. For the experiment described in Fig. 6a only, all three substrates were introduced into both cell lines in triplicate on the same day in parallel (then this was repeated on a second day), allowing us to explore relative joining efficiency when comparing different substrates. Joining efficiencies for Fig. 6a are thus expressed relative to that observed for undamaged 5′GATC after introduction into wild-type cells. Sequencing Template DNA for each sequencing library was pooled from the three independent electroporations performed on a single day. We amplified 5 × 10 5 input junction molecules (determined using qPCR) using Phusion DNA polymerase (NEB) and variants of the qPCR primers that have six-nucleotide barcode sequences appended to their 5′ ends for 21 cycles ( Supplementary Fig. 2c ). Amplified DNA (15.5 ng) from each amplified library was then pooled again in groups of 9–11 libraries (7 groups total), 5′ phosphorylated, treated to add dA to 3′ termini, and then ends further appended by ligation with an adaptor for paired-end sequencing (Illumina). Free adapter was removed by gel purification. A final pool of all gel purified libraries (109 separately indexed libraries for the run used here) was then amplified with adapter-specific primers for 10 cycles, purified (Agencourt Ampure XP, Beckman Coulter) and equal amounts (180 ng) of DNA from each group of libraries were combined and submitted for a 2 × 80 bp (that is, paired end run) sequencing run (MiSeq, Illumina) with a phiX174 DNA ‘spike-in’ to ensure matrix and phasing intensity calibration parameters could be accurately estimated. Reads with PhiX 174 DNA were removed. Paired-end reads were then merged and libraries de-indexed using Genomics workbench v6.0.3 (CLC-Bio). A proportion of improperly de-indexed reads in each library were identified by exact matches to the most frequent reads from other libraries and excluded, leaving 455,082 reads distributed over the 33 libraries (excluding controls) discussed here ( Supplementary Table 1 ). We assessed sample diversity after amplification using a control amplicon with an embedded degenerated tetramer, using the same input number of control amplicon molecules as experimental samples (5 × 10 5 ). We recovered all 256 sequence combinations of the degenerate tetramer in 18,883 reads, with representation of each sequence (number of reads for each sequence/total reads) distributed as shown ( Supplementary Fig. 2d ). Substitution error intrinsic to sample processing was assessed using another control library, prepared by in vitro ligation of 5′GATC substrate with T4-ligase. The mean substitution frequency over the length of this product was 1.2 × 10 −3 , ±9 × 10 −4 (s.d.). The frequency of single-nucleotide substitutions in reads from experimental samples was not significantly greater than the control, regardless of whether the position assessed was at the junction or in flanking DNA ( Supplementary Fig. 3b ). Analysis of experimental samples is thus restricted to counting exact matches to a test set of sequences that includes all combinations of terminal deletions from ends that can be both amplified by the primers described above, and distinguished as a unique sequence (this set comprises 165 sequences for AGCG3′; the number differs slightly for different substrates, according to variable presence of some sequence identities in the two flanks). We additionally included in the set junctions consistent with definitive ‘N-additions’ as identified by those reads with insertions of random length and sequence from intact ends. Notably, N-additions defined in this way were detected only when using 5′ overhang-containing substrates; even then, they were rare (<0.05% of recovered junctions), and almost exclusively observed after 5-h incubations in HCT-116 cells ( Supplementary Table 1 ). Finally, we compensated for reductions in the counts of reads of exact matches for each sequence due to processing-dependent substitution error according to the formula y = x (1−( a × n )), where y is the corrected count, x is the experimentally observed count of exact matches, a =1.2 × 10 −3 (average substitution frequency in control library) and n =length of tested sequence. Analysis of joining with G O termini G O -containing templates amplify less efficiently than undamaged templates ( Supplementary Fig. 2b ). Reduced amplification efficiency is thus expected to result in underestimation of retained G O by a factor of 2 as determined by both techniques described below. The frequency of A incorporation opposite G O (transversion mutation) during amplification was determined to be 89.0% under our sample preparation conditions, using a control library generated by in vitro ligation of the 5′G O ATC substrate with T4 DNA ligase. Retention of G O in junctions from cells was thus estimated by dividing observed transversion containing junctions by 0.89. The frequency of observed G containing junctions was then reduced by the difference between estimated G O and junctions with transversions. We also independently assessed presence of G O in junctions by probing the sensitivity of product to formamidopyrimidine [fapy]-DNA glycosylase (Fpg), an enzyme that incises at 8-oxoG ( Supplementary Fig. 4b,c ). We pre-digested qPCR reactions assembled as described above with 0.4 units of Fpg (New England BioLabs) for 1 h at 37 °C (or mock digested) before starting the standard qPCR cycling protocol. We defined the dynamic range of these assays using control T4 ligated GATC and G O ATC substrate. Control 5′ GATC-containing junctions were thus resistant to Fpg (112%, ±7, relative to undigested), while control G O ATC-containing junctions were sensitive (10.2%, ±0.1%, relative to undigested). This range was sufficient to confirm the majority of cellular G O ATC-containing junctions were fpg-sensitive, and this proportion decreases with time in the cell. However, the significant background resistance (10.2%) using pure model product indicates the low levels of Fpg-resistant product in our samples is a less accurate estimation of G O retention than is possible with sequencing analysis. In addition, this technique does not distinguish between the different causes for Fpg resistance (precise replacement with undamaged G, versus deletion of overhang). Interpretations in the results section thus focus on results of sequencing analysis. Statistical methods One-way analysis of variance (ANOVA) tests with P values adjusted by the Bonferonni method ( Fig. 6a ), or Student’s t -tests ( Supplementary Fig. 4a ), were used to compare the continuous variables between groups, as appropriate. Proportions of interest ( Supplementary Table 2 ) were compared via logistic regression models, with adjustment for extrabinomial variation as described [58] . This method allows and adjusts the estimates and the s.d.’s for variation that exceeds that of the binomial model. This extra variation can be due to correlation between the outcomes of the individual reads, each read being a classification, for example, into either direct or not. Analyses were performed using GraphPad Prism, GraphPad Software, San Diego, CA, USA and SAS version 9.2, Cary, NC, USA. How to cite this article: Waters, C. A. et al . The fidelity of the ligation step determines how ends are resolved during nonhomologous end joining. Nat. Commun. 5:4286 doi: 10.1038/ncomms5286 (2014).